WT1 interacts with MAD2 and regulates mitotic checkpoint function Tumour suppressors safeguard the fidelity of the mitotic checkpoint by transcriptional regulation of genes that encode components of the mitotic checkpoint complex (MCC). Here we report a new role for the tumour suppressor and transcription factor, WT1, in the mitotic checkpoint. We show that WT1 regulates the MCC by directly interacting with the spindle assembly checkpoint protein, MAD2. WT1 colocalizes with MAD2 during mitosis and preferentially binds to the functionally active, closed-conformer, C-MAD2. Furthermore, WT1 associates with the MCC containing MAD2, BUBR1 and CDC20, resulting in prolonged inhibition of the anaphase-promoting complex/cyclosome (APC/C) and delayed degradation of its substrates SECURIN and CYCLIN B1. Strikingly, RNA interference-mediated depletion of WT1 leads to enhanced turnover of SECURIN, decreased lag time to anaphase and defects in chromosome segregation. Our findings identify WT1 as a regulator of the mitotic checkpoint and chromosomal stability. WT1 is a zinc finger transcription factor that can activate or repress target genes that control cell growth and development [1] , [2] , [3] . WT1 is subject to alternative splicing in two regions: a 17-amino acid (aa) insertion within the central region of the protein (17AA) and the insertion of 3 aa (Lys-Thr-Ser) within the zinc finger region (KTS). WT1 is expressed in several organs and tissues of the embryo and is particularly important for the development of the urogenital system where it functions as a tumour suppressor [4] , [5] . Recent findings suggest that WT1 is a key regulator of mesenchyme to epithelial balance during development, and is also required for the maintenance of several adult tissues [6] . A considerable body of evidence suggests that WT1 can also act as an oncogene [7] , [8] . WT1 is overexpressed in several cancers, including leukemia, breast, ovary, bone, lung and brain, and is a promising therapeutic target [9] , [10] . The accuracy of cell division is monitored at several steps and is initiated at the beginning of mitosis by the spindle assembly checkpoint (SAC). The SAC components, which include MAD1, MAD2, BUBR1 and BUB3, play key roles to ensure correct attachment of chromosomes to the mitotic spindle and fidelity of chromosomal segregation during cell division. Impaired SAC function promotes aneuploidy and contributes to genomic instabilities and tumorigenesis [11] , [12] , [13] . Indeed, a majority of human tumours accumulate mutations that deregulate the expression of proteins essential for mitotic checkpoint function [14] , [15] , [16] . This results in missegregation of chromosomes during mitosis and contributes to chromosome instability (CIN). MAD2 adopts two native conformations, open (O-MAD2) and closed (C-MAD2), and has the ability to self-dimerize. C-MAD2 is the functionally active form of MAD2, which engages in the formation and maintenance of the checkpoint signal cascade [17] , [18] , [19] , [20] . The presence of unattached kinetochores activates the SAC signal in which the MAD2–MAD1 complex generates a diffusible anaphase wait signal. This mitotic checkpoint complex (MCC) composed of MAD2, BUBR1, CDC20 and BUB3 then inhibits the anaphase-promoting complex/cyclosome (APC/C). The ubiquitin ligase activity of APC/C is critical for the degradation of SECURIN and CYCLIN B1, and eventual anaphase entry [12] , [21] , [22] , [23] , [24] , [25] . Several lines of evidence suggest that human tumours with CIN have misregulated expression of MAD2. Studies in mice heterozygous for MAD2 showed increased frequency towards aneuploidy [26] , [27] , [28] . Here we show that WT1 associates with C-MAD2 during mitosis and regulates the mitotic checkpoint function. We demonstrate that through interaction with MAD2, WT1 inhibits APC/C-mediated degradation of SECURIN and CYCLIN B1, and that ablation of WT1 protein in cells that normally express WT1 leads to chromosomal-segregation defects and early anaphase entry. Our results reveal a previously unknown role of WT1 in the direct regulation of mitotic checkpoint function and genomic stability via its interaction with MAD2. WT1 interacts with MAD2 during mitosis A yeast two-hybrid screen performed with a discrete region of mouse WT1 protein (residues 245–297; that contains the 17AA) using a HeLa complementary DNA library revealed MAD2 as a potential interaction partner. A direct interaction between WT1 and MAD2 was confirmed in vitro by glutathione S -transferase (GST)-pulldown assay where recombinant full-length (FL) His-tagged MAD2 protein associated with GST-WT1 (245–297) but not with the control GST beads ( Fig. 1a ). Furthermore, Flag-tagged FL human WT1 protein was also found to interact with MAD2 in vitro ( Fig. 1b ). Binding assays comparing GST-WT1+17AA (residues 180–297) and GST-WT1 Δ17AA (lacking the 17AA) revealed that the 17AA region of WT1 was dispensable for the MAD2 interaction ( Fig. 1c ). 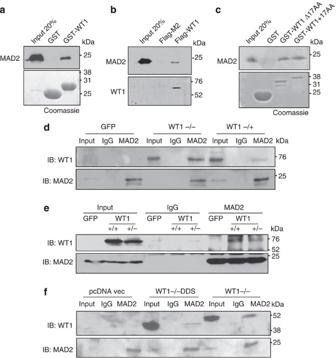Figure 1: WT1 interacts with MAD2. (a)In vitrointeraction assay was performed with either GST-WT1 (residues 245–297) or GST in the presence of FL His-MAD2. The interaction was analysed by immunoblotting with anti-MAD2 antibody. Bound proteins were also resolved by SDS–PAGE and stained with Coomassie Brilliant Blue. (b)In vitropull-down assay was also performed with either Flag-M2 magnetic beads alone or incubated with FL Flag-tagged WT1 protein in the presence of His-MAD2. The interaction was analysed by immunoblotting with anti-WT1 and anti-MAD2 antibodies. (c) GST interaction assay was carried out with WT1 containing the 17 aa insertion (residues 180–297, +17AA) or lacking it (residues 180–297, Δ17AA) with His-MAD2. The interaction was analysed by immunoblotting with anti-MAD2 antibody. Bound proteins were also resolved by SDS–PAGE and stained with Coomassie Brilliant Blue. (d) HeLa cells were transfected with GFP Vector, FL GFP-WT1 (−/−) or GFP-WT1 (−/+) isoforms, and 48 h later whole-cell extracts were prepared, followed by immunoprecipitation with anti-MAD2 antibodies. The immunoprecipitates were probed with anti-WT1 antibody. Blotting with anti-MAD2 antibody was performed as a control. (e) The MAD2 interaction with ectopically expressed GFP-tagged FL WT1 (+/+) and WT1 (+/−) isoforms was analysed as ind(f) HeLa cells were transfected with pcDNA vector, pcDNA driving expression of WT1−/−DDS (R394X) or wild-type WT1−/−, followed by immunoprecipitation with anti-MAD2 antibodies. The immunoprecipitates were probed with anti-WT1 antibodies. Blotting with anti-MAD2 antibodies was performed as a control. Figure 1: WT1 interacts with MAD2. ( a ) In vitro interaction assay was performed with either GST-WT1 (residues 245–297) or GST in the presence of FL His-MAD2. The interaction was analysed by immunoblotting with anti-MAD2 antibody. Bound proteins were also resolved by SDS–PAGE and stained with Coomassie Brilliant Blue. ( b ) In vitro pull-down assay was also performed with either Flag-M2 magnetic beads alone or incubated with FL Flag-tagged WT1 protein in the presence of His-MAD2. The interaction was analysed by immunoblotting with anti-WT1 and anti-MAD2 antibodies. ( c ) GST interaction assay was carried out with WT1 containing the 17 aa insertion (residues 180–297, +17AA) or lacking it (residues 180–297, Δ17AA) with His-MAD2. The interaction was analysed by immunoblotting with anti-MAD2 antibody. Bound proteins were also resolved by SDS–PAGE and stained with Coomassie Brilliant Blue. ( d ) HeLa cells were transfected with GFP Vector, FL GFP-WT1 (−/−) or GFP-WT1 (−/+) isoforms, and 48 h later whole-cell extracts were prepared, followed by immunoprecipitation with anti-MAD2 antibodies. The immunoprecipitates were probed with anti-WT1 antibody. Blotting with anti-MAD2 antibody was performed as a control. ( e ) The MAD2 interaction with ectopically expressed GFP-tagged FL WT1 (+/+) and WT1 (+/−) isoforms was analysed as in d ( f ) HeLa cells were transfected with pcDNA vector, pcDNA driving expression of WT1−/−DDS (R394X) or wild-type WT1−/−, followed by immunoprecipitation with anti-MAD2 antibodies. The immunoprecipitates were probed with anti-WT1 antibodies. Blotting with anti-MAD2 antibodies was performed as a control. Full size image We next sought to determine whether MAD2 interacts with all the four major isoforms of human WT1 in the cells. HeLa cells (which do not express WT1) were transfected with a plasmid driving expression of either green fluorescent protein (GFP), GFP linked to FL WT1 (−/− isoform, which does not contain either the 17AA or KTS insertions) or FL GFP-tagged WT1 (−/+ isoform, which lacks the 17AA but contains the KTS insertion). Whole-cell extracts were prepared and MAD2 immunoprecipitates from the transfected cells were analysed by immunoblotting with anti-WT1 antibodies, which confirmed that both the −/− and −/+ WT1 isoforms interact with endogenous MAD2 ( Fig. 1d ). Similar interaction assays were carried out with the other FL GFP-tagged WT1 isoforms, the WT1 (+/+) that contains both the 17AA and the KTS regions, and WT1 (+/−) that contains the 17AA but not the KTS domain ( Fig. 1e ). The results showed that endogenous MAD2 could interact with all four major isoforms of WT1. We also analysed a WT1 mutant derivative (R394X) that mimics those found in Denys Drash syndrome (WT1 −/−DDS) and lacks an intact DNA-binding domain. The results revealed a weaker MAD2-binding efficiency of WT1 −/−DDS with respect to FL WT1 −/− ( Fig. 1f ), suggesting that DNA binding might play a role in bringing WT1 in close proximity to MAD2. To determine the MAD2-binding domain of WT1, several internal deletion mutants of GST-WT1 were generated ( Fig. 2a , schematic) and tested for their ability to interact with MAD2. Deletion of the region between residues 280 and 295 (Δ3 and Δ4) led to a significant reduction in the WT1-MAD2 interaction ( Fig. 2a ). We therefore deleted the (Δ4) region spanning amino acids 288–295 in the FL human GFP-WT1−/− isoform and tested whether this region of WT1 is crucial for MAD2 interaction in cells. The results showed significant reduction in GFP-WT1−/−Δ4 and MAD2 interaction when compared with GFP-WT1−/− ( Fig. 2b ). 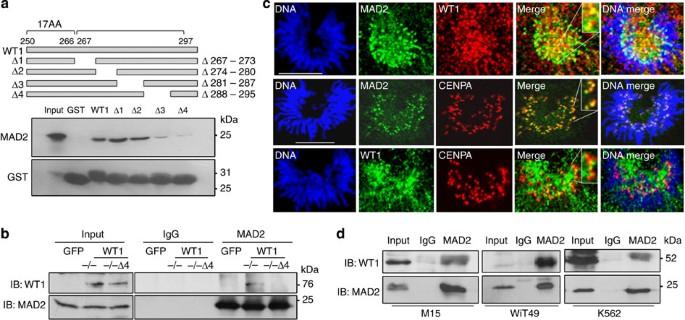Figure 2: Endogenous WT1 interacts with MAD2. (a) GST interaction assays were performed with the internal deletion mutants of GST-WT1 (schematic) with FL His-MAD2 and immunoblotted with anti-MAD2 and anti-GST antibodies. (b) Co-immunoprecipitation assays were carried out with whole-cell extracts derived from HeLa cells that had been transfected with either GFP vector, GFP WT1 (−/−) or GFP-WT1 (−/−Δ4) using anti-MAD2 or anti-WT1 antibodies. (c) Co-immunofluorescence analysis was carried out in WiT49 cells with anti-MAD2 and anti-WT1 antibodies at the pro-metaphase stage of mitosis. DNA was stained with Hoechst. Scale bar, 10 μm. (d) M15, WiT49 and K562 cells were treated with 60 ng ml−1nocodazole for 24 h, whole-cell extracts prepared and immunoprecipitation performed with anti-MAD2 antibodies followed by immunoblotting with WT1 antibody. Input is 10% of the total whole-cell extract. Figure 2: Endogenous WT1 interacts with MAD2. ( a ) GST interaction assays were performed with the internal deletion mutants of GST-WT1 (schematic) with FL His-MAD2 and immunoblotted with anti-MAD2 and anti-GST antibodies. ( b ) Co-immunoprecipitation assays were carried out with whole-cell extracts derived from HeLa cells that had been transfected with either GFP vector, GFP WT1 (−/−) or GFP-WT1 (−/−Δ4) using anti-MAD2 or anti-WT1 antibodies. ( c ) Co-immunofluorescence analysis was carried out in WiT49 cells with anti-MAD2 and anti-WT1 antibodies at the pro-metaphase stage of mitosis. DNA was stained with Hoechst. Scale bar, 10 μm. ( d ) M15, WiT49 and K562 cells were treated with 60 ng ml −1 nocodazole for 24 h, whole-cell extracts prepared and immunoprecipitation performed with anti-MAD2 antibodies followed by immunoblotting with WT1 antibody. Input is 10% of the total whole-cell extract. Full size image We next performed co-immunofluorescence analysis in WiT49 cells (a Wilms’ tumour-derived cell line that expresses endogenous wild-type WT1) with anti-MAD2 and anti-WT1 antibodies, which revealed a significant co-localization pattern during the pro-metaphase of mitosis ( Fig. 2c ). The centromeric localization of MAD2 and WT1 was also studied using anti-CENPA antibodies in our colocalization assays. MAD2 and CENPA were juxtaposed close to the centromeres, while WT1 was localized at the surrounding regions of the centromeres. To study the association between endogenous WT1 and MAD2 during activation of the checkpoint, co-immunoprecipitation analysis was performed with whole-cell extracts prepared from nocodazole-treated M15 cells (mouse mesonephric cell line), WiT49 cells (human Wilms’ tumour cell line) and K562 cells (derived from human chronic myelogenous leukemia). In each case, the endogenous WT1 was present in MAD2 immunoprecipitates ( Fig. 2d ). These results raised the possibility that the association of WT1 with MAD2 might play a role in the regulation of SAC function. WT1 interacts with the active closed MAD2 conformer MAD2 protein can adopt two native conformations: the closed (C-MAD2) or the open (O-MAD2) conformers [17] , [18] , [19] , [20] . At the onset of mitosis, O-MAD2 is recruited to the unattached kinetochores of the pro-metaphase chromosomes with the help of its partner MAD1, which catalyses the conversion of O-MAD2 to C-MAD2 conformer. The MAD1-C-MAD2 tetramer acts as a template for additional O- to C-MAD2 conversion and initiates active SAC signalling. CDC20 is a critical C-MAD2-binding partner, which occupies the same binding site on MAD2 as MAD1. Binding of either MAD1 or CDC20 facilitates the formation of the C-MAD2 conformation [29] , [30] . A 12-aa MAD2-binding peptide (MBP1) has been generated that competes for the same site on MAD2 that is bound by MAD1 or CDC20. Comparative nuclear magnetic resonance and co-crystal studies have revealed that the MAD2-MBP1 complex adopts the C-MAD2 conformation, mimicking MAD2 structure in either the MAD2–MAD1 or MAD2–CDC20 complexes [18] , [29] . We therefore employed MBP1 in our interaction studies to test the binding preference of WT1 with the MAD2 conformers. Recombinant wild-type MAD2 protein equilibrates between O- and C-MAD2 conformers and incubation of MAD2 with MBP1 shifts the equilibrium towards C-MAD2 conformer. Pull-down assays were carried out with GST-WT1 (245–297) and MAD2 that had been pre-incubated with either MBP1, or a control peptide. The data revealed that GST-WT1 (245–297) has a higher affinity for MAD2 that was pre-bound to MBP1 and therefore for C-MAD2 ( Fig. 3a ). 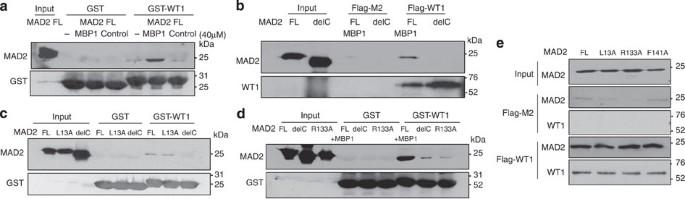Figure 3: WT1 has higher affinity for the active closed MAD2 conformer. (a) GST interaction assays were carried out with WT1 (residues 245–297) and FL His-MAD2 alone, and also with MAD2 pre-incubated with either 40 μM of MBP1, or a control peptide. The pull-down complexes were resolved by SDS–PAGE and immunoblotted with anti-MAD2 antibodies. (b)In vitropull-down assays were performed with either Flag-M2 magnetic beads alone or FL Flag-tagged WT1 protein in the presence of FL His-MAD2 (pre-incubated with MBP1) or the MAD2 delC mutant. The interaction was analysed by immunoblotting with anti-WT1 and anti-MAD2 antibodies. (c) GST interaction assays were carried out with His-MAD2, MAD2 L13A and MAD2-C-terminal deletion mutant (Del-C). Immunoblotting was performed using anti-MAD2 and anti- GST antibodies. (d) GST interaction assays were carried out with His-MAD2+MBP1, MAD2-Del-C and MAD2 dimerization mutant, R133A. Immunoblotting was performed using anti-MAD2 and anti-GST antibodies. (e) Pull-down assays were performed with FL Flag-WT1 protein and the different MAD2 point mutant derivatives. Immunoblotting was performed using anti-MAD2 and anti-WT1 antibodies. Input is 20% of the different MAD2 proteins used for interaction analysis. Figure 3: WT1 has higher affinity for the active closed MAD2 conformer. ( a ) GST interaction assays were carried out with WT1 (residues 245–297) and FL His-MAD2 alone, and also with MAD2 pre-incubated with either 40 μM of MBP1, or a control peptide. The pull-down complexes were resolved by SDS–PAGE and immunoblotted with anti-MAD2 antibodies. ( b ) In vitro pull-down assays were performed with either Flag-M2 magnetic beads alone or FL Flag-tagged WT1 protein in the presence of FL His-MAD2 (pre-incubated with MBP1) or the MAD2 delC mutant. The interaction was analysed by immunoblotting with anti-WT1 and anti-MAD2 antibodies. ( c ) GST interaction assays were carried out with His-MAD2, MAD2 L13A and MAD2-C-terminal deletion mutant (Del-C). Immunoblotting was performed using anti-MAD2 and anti- GST antibodies. ( d ) GST interaction assays were carried out with His-MAD2+MBP1, MAD2-Del-C and MAD2 dimerization mutant, R133A. Immunoblotting was performed using anti-MAD2 and anti-GST antibodies. ( e ) Pull-down assays were performed with FL Flag-WT1 protein and the different MAD2 point mutant derivatives. Immunoblotting was performed using anti-MAD2 and anti-WT1 antibodies. Input is 20% of the different MAD2 proteins used for interaction analysis. Full size image Studies with several deletion and point mutants of MAD2 have identified residues that are important for its dimerization and also for acquiring the C/O-MAD2 state [18] , [31] . Deletion of 10 aa at the carboxy terminus results in a MAD2 derivative that is locked in the O-conformation and cannot bind MAD1, CDC20 or MBP1 (ref. 31 ). Similarly, when MAD2 lysine residue 13 is substituted to alanine (L13A), it results in a MAD2 derivative locked in C-conformation, while substitution of arginine residue 133 with alanine (R133A) generates the monomeric form of MAD2, which cannot self-dimerize. We generated a C-terminal 10 aa deletion mutant of MAD2 (Del-C), C-MAD2 mutant (L13A) and MAD2 dimerization mutant, R133A and F141A, and then compared their ability to interact with WT1 with respect to MBP1-bound C-MAD2. We performed pull-down assays with FL MAD2 (pre-incubated with MBP1 to generate C-MAD2) and MAD2 Del-C mutant (O-MAD2) in the presence of either Flag-M2 beads or Flag-tagged FL WT1 protein. Interestingly, FL WT1 showed a greater level of binding to MAD2 that was pre-incubated with MBP1, suggesting that WT1 has a higher affinity to interact with C-MAD2 ( Fig. 3b ). Furthermore, GST-pull-down assays showed that WT1 (residues 245–297) has higher affinity to interact with C-MAD2 (L13A) when compared with MAD2 Del-C ( Fig. 3c ). WT1 can also bind to O-MAD2 (Del-C), but at a lower affinity than that observed for C-MAD2 that is induced by MBP1 ( Fig. 3d ). The different structural mutants of MAD2 (L13A, R133A and F141A) were also found to efficiently interact with FL Flag-WT1 ( Fig. 3e ). Taken together, these results suggest that WT1 binds preferentially to C-MAD2 and that WT1 does not bind to the same site in MAD2 as either MAD1 or CDC20. To test whether WT1 can form a complex with MAD2 along with other components of the MCC, we induced the spindle checkpoint in K562 cells with nocodazole or taxol, prepared whole-cell extracts and immunoprecipitated either MAD2 or WT1 followed by immunoblotting with anti-BUBR1, MAD1, CDC20, WT1 and MAD2 antibodies ( Fig. 4a ). Both anti-WT1 and anti-MAD2 antibodies co-immunoprecipitated MAD1, CDC20 and BUBR1, suggesting that WT1 can associate with activated spindle/MCCs. The association of WT1 with the MAD2–MAD1 complex is consistent with its localization during the pro-metaphase stage (as seen in Fig. 2c ). We therefore determined the effect of MAD2 depletion on the subcellular localization of WT1 during pro-metaphase. Co-immunofluorescence analysis of WT1 and MAD2 was performed in WiT49 cells that had been transfected with MAD2 small interfering RNA (siRNA), which resulted in the loss of WT1 localization pattern at the chromosomes when compared with cells transfected with control siRNA ( Fig. 4b,c ). Comparable effects were seen when we performed a similar experiment in M15 cells ( Supplementary Fig. 1 ). However, RNA interference-mediated depletion of WT1 did not adversely affect the localization of MAD2 ( Fig. 4b and Supplementary Fig. 1 ). Taken together, these results show that WT1 associates with the active C-MAD2 complex during mitosis, suggesting a potential role in MAD2-dependent checkpoint functions. 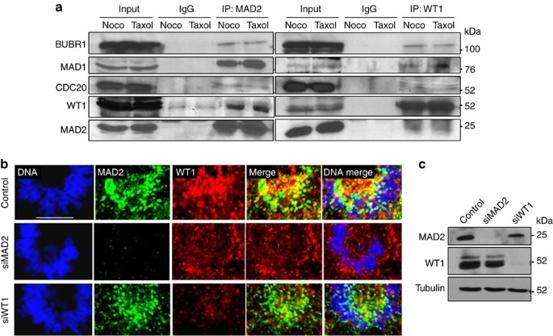Figure 4: WT1 interacts with the MCC. (a) K562 cells were treated with 60 ng ml−1of either nocodazole or taxol. MAD2 and WT1 immunoprecipitates were analysed by immunoblotting with the indicated antibodies. Input is 10% of the total whole-cell extract used for immunoprecipitations. (b) WiT49 cells were transfected with control, MAD2 siRNA or WT1 siRNA for 48 h, followed by immunofluorescence analysis with anti-MAD2 and anti-WT1 antibodies in the pro-metaphase stage of mitosis. DNA was stained with Hoechst. Scale bar, 10 μm. (c) Immunoblotting was performed with anti-MAD2, anti-WT1 and anti-TUBULIN antibodies for control and MAD2, or WT1 siRNA-transfected cells. Figure 4: WT1 interacts with the MCC. ( a ) K562 cells were treated with 60 ng ml −1 of either nocodazole or taxol. MAD2 and WT1 immunoprecipitates were analysed by immunoblotting with the indicated antibodies. Input is 10% of the total whole-cell extract used for immunoprecipitations. ( b ) WiT49 cells were transfected with control, MAD2 siRNA or WT1 siRNA for 48 h, followed by immunofluorescence analysis with anti-MAD2 and anti-WT1 antibodies in the pro-metaphase stage of mitosis. DNA was stained with Hoechst. Scale bar, 10 μm. ( c ) Immunoblotting was performed with anti-MAD2, anti-WT1 and anti-TUBULIN antibodies for control and MAD2, or WT1 siRNA-transfected cells. Full size image WT1 inhibits APC/C function Our data so far suggest that WT1 associates with C-MAD2 that forms part of the MCC. An essential function of the MCC is to inhibit APC/C, an E3-ubiquitin ligase that marks SECURIN and CYCLIN B1 for degradation, leading to chromosomal separation during anaphase. To determine whether WT1 plays a role in the regulation of MAD2-dependent APC/C inhibition, a ubiquitination/degradation assay was performed with mitotic extracts prepared from nocodazole-arrested HeLa cells (which do not express WT1), to which we added either GST or GST-WT1, and incubated for different time periods. The results showed that GST-WT1 significantly delayed the degradation of SECURIN and CYCLIN B1 by APC/C compared with GST ( Fig. 5a ). Immunoblotting with anti-MAD2, GST and CDC27 (a subunit of APC/C) antibodies was performed as controls. Quantitation of the levels of SECURIN and CYCLIN B1 at the 45 min time point are plotted as graphs ( Fig. 5b ). The GST-WT1-Δ4 mutant (MAD2-interaction-defective mutant lacking residues 288–295; see Fig. 2a ) did not delay SECURIN and CYCLIN B1 degradation, confirming that direct association with MAD2 is essential for WT1-mediated APC/C inhibition ( Fig. 5c ). 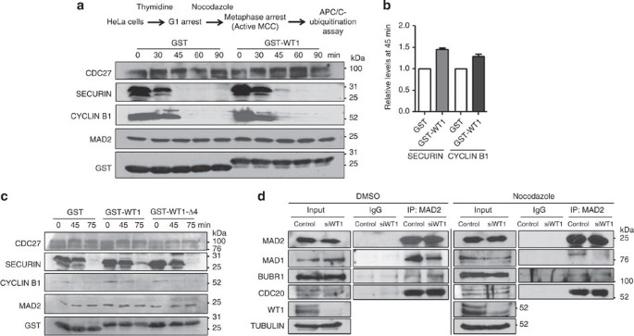Figure 5: WT1 inhibits APC/C function. (a) APC/C ubiquitination assay was performed with mitotic extracts derived from nocodazole-arrested HeLa cells in the presence of GST control or GST-WT1 (residues 245–297) for different time periods. The reaction was stopped at 0, 30, 45, 60 and 90 min, and immunoblotting was performed with the indicated antibodies. The degradation of SECURIN and CYCLIN B1 was monitored for the indicated time points. (b) The band intensity at 45 min time point for SECURIN and CYCLIN B1 degradation in the presence of GST control or GST-WT1 from three independent experiments was quantified using Image J software and plotted graphically. Error bars are s.d. from the mean. (c) APC/C ubiquitination assay was performed as ina, with GST, GST-WT1 (residues 245–297) and GST-WT1Δ4 (Δ 288–295) at different time points and immunoblotted with the antibodies indicated. (d) WiT49 cells were transfected with either control or WT1 siRNA for 48 h, followed by treating the cells with either DMSO or nocodazole (60 ng ml−1) for a further 12 h. Whole-cell extracts were prepared and MAD2 was immunoprecipitated then immunoblotted with anti-MAD1, anti-BUBR1, anti-CDC20 and anti-MAD2 antibodies. Input is 10% of the total whole-cell extract used for immunoprecipitation. Figure 5: WT1 inhibits APC/C function. ( a ) APC/C ubiquitination assay was performed with mitotic extracts derived from nocodazole-arrested HeLa cells in the presence of GST control or GST-WT1 (residues 245–297) for different time periods. The reaction was stopped at 0, 30, 45, 60 and 90 min, and immunoblotting was performed with the indicated antibodies. The degradation of SECURIN and CYCLIN B1 was monitored for the indicated time points. ( b ) The band intensity at 45 min time point for SECURIN and CYCLIN B1 degradation in the presence of GST control or GST-WT1 from three independent experiments was quantified using Image J software and plotted graphically. Error bars are s.d. from the mean. ( c ) APC/C ubiquitination assay was performed as in a , with GST, GST-WT1 (residues 245–297) and GST-WT1Δ4 (Δ 288–295) at different time points and immunoblotted with the antibodies indicated. ( d ) WiT49 cells were transfected with either control or WT1 siRNA for 48 h, followed by treating the cells with either DMSO or nocodazole (60 ng ml −1 ) for a further 12 h. Whole-cell extracts were prepared and MAD2 was immunoprecipitated then immunoblotted with anti-MAD1, anti-BUBR1, anti-CDC20 and anti-MAD2 antibodies. Input is 10% of the total whole-cell extract used for immunoprecipitation. Full size image To study the possible mechanism by which WT1 inhibits APC/C activity, co-immunoprecipitation analysis was carried out with whole cell extracts derived from WiT49 cells that had been transfected with either control or WT1 siRNA followed by treatment with dimethyl sulphoxide (DMSO) or nocodazole (60 ng ml −1 ). The results showed that on WT1 silencing the association of MAD2 with MAD1 was significantly reduced in both DMSO as well as nocodazole-treated cells ( Fig. 5d ), suggesting a potential role of WT1 in promoting MAD2–MAD1 interaction during the initiation of active checkpoint signalling. Thus, WT1 integrates with and enhances the formation of MAD2-containing spindle/MCCs, leading to a sustained inhibition of APC/C activity. The results also show that WT1 does not compete with MAD1 for MAD2 binding. Presumably, WT1 may promote the stability of MAD1–MAD2 tetramer or recruit more O-MAD2 for amplifying the SAC signal. Alternatively, WT1 could also induce or stabilize C-MAD2 conformation. Structural insights from MAD2-WT1 association would reveal more information regarding the mode of action of WT1 during checkpoint activation. Depletion of WT1 promotes mitotic segregation defects Our results show that the interaction between WT1 and MAD2 enhances MCC function and leads to prolonged inhibition of APC/C activity. This suggests that stimulation of SAC function by WT1 could potentially affect chromosomal stability and genomic integrity. To test this possibility, WiT49 cells were treated with control siRNA, WT1 siRNA or MAD2 siRNA for 48 h, followed by immunofluorescence analysis using anti-WT1 antibodies ( Fig. 6a ). Depletion of WT1 protein resulted in an enhanced rate of chromosome lagging and bridges during anaphase, which was strikingly similar to the defects observed on MAD2 silencing in WiT49 cells ( Fig. 6a , compare central two panels with lower panel). Quantitation of lagging chromosomes in control and WT1 siRNA-transfected WiT49 cells is shown in Fig. 6b . Transfection of M15 cells with WT1 siRNA also caused a significant increase in lagging chromosomes ( Fig. 6b ). Consistent with these observations, siRNA-mediated knockdown of either WT1 or MAD2 resulted in faster degradation of SECURIN when compared with control siRNA in WiT49 cells treated with either DMSO or nocodazole ( Fig. 6c ). 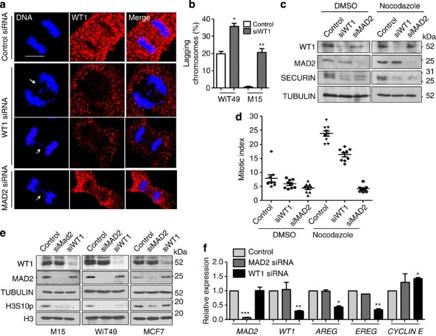Figure 6: WT1 knockdown increases the rate of mitotic abnormalities. (a) WiT49 cells were transfected with control, WT1, or MAD2 siRNA, and 48 h later immunofluorescence analysis was performed with anti-WT1 antibodies to study the anaphase stage of mitosis. DNA was stained with Hoechst. Scale bar, 10 μm. (b) The percentage of WiT49 and M15 cells exhibiting mitotic defects (chromosome lagging/bridges) was scored over total number of cells that were in anaphase for >100 optical fields and plotted graphically. Error bars are s.d. from the mean for three independent experiments, and statistical significance was determined by Student’st-test (P<0.05). (c) WiT49 cells were transfected with control, WT1 or MAD2 siRNAs for 48 h followed by treatment with either DMSO or nocodazole (60 ng ml−1) for another 24 h. Whole-cell extracts were prepared and immunoblotted with anti-WT1, MAD2, SECURIN and TUBULIN antibodies (d) Mitotic indices were calculated for WiT49 cells transfected with control, WT1 or MAD2 siRNA, followed by DMSO or nocodazole (60 ng ml−1) treatment. The results were plotted as graphs after analysing >100 optical fields for at least three independent experiments. Error bars are s.d. from the mean. (e) M15, WiT49 and MCF7 cells were transfected with control, MAD2 or WT1 siRNAs for 48 h followed by immunoblotting with anti-WT1, anti-MAD2, anti-TUBULIN, anti-phosphorylated Histone H3 serine10 (H3S10p) and anti-Histone H3 antibodies. (f) Quantitative RT–PCR analysis was performed to analyse the expression ofMAD2,WT1,AREG,EREGandCYCLIN Egenes in WiT49 cells transfected with control, MAD2 siRNA or WT1 siRNA for 48 h. Error bars denote s.d. from the mean of three independent experiments and statistical significance was analysed by Student’st-test (P<0.05). Figure 6: WT1 knockdown increases the rate of mitotic abnormalities. ( a ) WiT49 cells were transfected with control, WT1, or MAD2 siRNA, and 48 h later immunofluorescence analysis was performed with anti-WT1 antibodies to study the anaphase stage of mitosis. DNA was stained with Hoechst. Scale bar, 10 μm. ( b ) The percentage of WiT49 and M15 cells exhibiting mitotic defects (chromosome lagging/bridges) was scored over total number of cells that were in anaphase for >100 optical fields and plotted graphically. Error bars are s.d. from the mean for three independent experiments, and statistical significance was determined by Student’s t -test ( P <0.05). ( c ) WiT49 cells were transfected with control, WT1 or MAD2 siRNAs for 48 h followed by treatment with either DMSO or nocodazole (60 ng ml −1 ) for another 24 h. Whole-cell extracts were prepared and immunoblotted with anti-WT1, MAD2, SECURIN and TUBULIN antibodies ( d ) Mitotic indices were calculated for WiT49 cells transfected with control, WT1 or MAD2 siRNA, followed by DMSO or nocodazole (60 ng ml −1 ) treatment. The results were plotted as graphs after analysing >100 optical fields for at least three independent experiments. Error bars are s.d. from the mean. ( e ) M15, WiT49 and MCF7 cells were transfected with control, MAD2 or WT1 siRNAs for 48 h followed by immunoblotting with anti-WT1, anti-MAD2, anti-TUBULIN, anti-phosphorylated Histone H3 serine10 (H3S10p) and anti-Histone H3 antibodies. ( f ) Quantitative RT–PCR analysis was performed to analyse the expression of MAD2 , WT1 , AREG , EREG and CYCLIN E genes in WiT49 cells transfected with control, MAD2 siRNA or WT1 siRNA for 48 h. Error bars denote s.d. from the mean of three independent experiments and statistical significance was analysed by Student’s t -test ( P <0.05). Full size image Ablation of MAD2 protein results in defective SAC signalling. As a consequence, cells exit mitosis without stringent monitoring of kinetochore-spindle attachment errors. We scored the relative mitotic indices for WiT49 cells transfected with control, MAD2 or WT1 siRNAs ( Fig. 6d ). The mitotic index was drastically reduced on MAD2 silencing in nocodazole-treated cells. Knockdown of WT1 also showed significant reduction in the number of metaphase cells in nocodazole-treated cells when compared with control. These results suggest that the absence of either MAD2 or WT1 abrogates SAC function, leading to faster exit from mitosis and accumulation of chromosome-segregation defects in the cells. We also determined whether chromatin condensation during mitosis was affected on MAD2 or WT1 silencing. Interestingly, we observed a large reduction in the level of Histone H3 serine10 phosphorylation (H3S10p) in WiT49 and M15 cells transfected with either MAD2 or WT1 siRNAs ( Fig. 6e ). However, the effect of WT1 knockdown was not significant in MCF7 cells, suggesting the possible role of other cell-type-specific components in the regulation of WT1 functions during mitosis. Taken together, the data in Fig. 6a–e suggest that loss of WT1 results in a hypo-active SAC signalling and early anaphase entry, leading to an increase in erroneous or incomplete spindle attachments to the kinetochores and chromosome lagging during anaphase. WT1 is a transcription factor with diverse functions in the cell ranging from organogenesis and tumour suppression to oncogenesis [6] , [7] , [8] , [9] , [10] , [32] . In this study we have uncovered a unique role for WT1 as a mitotic checkpoint regulator. WT1 performs this function without significantly affecting the expression of genes crucial for SAC/MCC regulation. We also found that depletion of MAD2 by siRNA does not influence transcription of WT1 target genes ( Fig. 6f ). Several transcription factors are known to regulate the mitotic checkpoint through control of the expression of SAC and MCC components [33] . Our finding of a direct role for WT1 in the MCC has demonstrated a novel mechanism of action for a tumour suppressor/oncogene in the control of mitosis. WT1 is aberrantly expressed in tumours of several different origins [7] , [9] , [10] . Thus, a role in the regulation of APC/C activity could potentially contribute to the misregulation of the mitotic checkpoint in tumorigenesis. Conversely, loss of WT1 protein could compromise the SAC function, and thereby contribute to increased mitotic checkpoint failure and eventually CIN. Indeed, loss of WT1 has also been associated with abnormal chromosome number [34] , [35] . It would be of interest to study whether aberrant WT1 expression contributes to aneuploidy in different cancers as an outcome of its role in the regulation of cell cycle checkpoint. There are several factors that modulate MAD2-dependent checkpoint functions. p31 comet is a critical regulator of MAD2, which interacts with MAD1- or CDC20-bound MAD2 and negatively regulates the SAC function. p31 comet binds to the dimerization interface of MAD2 and promotes dissociation of CDC20-MAD2 containing MCC [36] , [37] . Interestingly, WT1 influences MAD2 function in an opposite manner to p31 comet and instead stabilizes MCC-mediated inhibition of APC/C and positively regulates the SAC function. WT1 preferentially binds to MBP1-bound MAD2, suggesting it favours the C-MAD2 conformer and does not compete with either MAD1 or CDC20 binding. Furthermore, knockdown of WT1 reduces MAD1–MAD2 interaction in the cells, which indicate that WT1 is not a competitive inhibitor of MAD1. Rather it augments MAD1–MAD2 association crucial for active SAC signalling. This property of WT1 is also different from the role played by Shugoshin (human Sgo2), which competes with MAD1 and CDC20 for binding to MAD2 during meiosis [38] . WT1 neither competes with MAD2-dimerization interface nor the MAD1/CDC20-binding site, yet significantly influences MAD2-dependent MCC functions. The interplay among these cellular regulators of MAD2 and their relative expression could therefore influence the final timing of anaphase entry and stringency of chromosome segregation. Our findings also raise the likelihood that other tumour suppressors might also act on the MCC directly and not only through the regulation of the abundance of MCC components. Cell culture and transfection WiT49 (derived from human anaplastic Wilms’ tumour), HeLa (derived from human cervical carcinoma), MCF7 (derived from human breast ductal carcinoma) and M15 (derived from developing mouse kidney) cells were grown in DMEM, and K562 cells (derived from chronic myelogenous leukemia) were grown in RPMI, supplemented with 10% (vol/vol) fetal bovine serum at 37 °C. Transfection of plasmids was performed using Effectene reagent (Qiagen). Cells were harvested 48 h after transfection and processed for different assays. The human and mouse MAD2 siRNAs and mouse WT1 siRNA were obtained from Qiagen. Human WT1 siRNA was obtained from Ambion. siRNAs were transfected using Hiperfect reagent (Qiagen) for 48 h. Plasmid constructs and protein purification FL human MAD2 was cloned from HeLa cDNA library in PRSET-A His-tagged vector. Point and deletion mutants were generated using a site-directed mutagenesis kit (Agilent). GST, GST-WT1 (and deletion mutants) were expressed in BL21-DE3 competent cells, and His-tagged human MAD2 (and mutant derivatives) were expressed in BL21-DE3(pLysS) competent cells followed by affinity purification as described before [39] . Flag-tagged FL WT1 protein (residue 1–449, including exon 5/17AA and KTS) was purchased from Creative Biomart. The MBP1 was purchased from Peptide 2.0 (sequence: SWYSYPPPQRAV); Control peptide sequence: CKATKDPSRVGDS. GFP-tagged FL isoforms WT1 (−/−) and WT1 (−/+) were kind gifts from Professor Brigitte Royer-Pokora. GFP-tagged FL isoform WT1 (+/+) was purchased from GeneCopoeia Inc., and GFP WT1 (+/−) was generated by deleting the KTS region using site-directed mutagenesis kit (Agilent). RNA analysis Total RNA was prepared using the QIAGEN RNeasy kit and cDNA was prepared using the BioRad iScript cDNA synthesis kit. Real-time PCR was performed using a BioRad MiniOpticon System and BioRAd SYBR Green assay reagents. Primers used in the analysis were: MAD2 , Fwd: 5′- ACGGTGACATTTCTGCCACT -3′, Rev: 5′- TGGTCCCGACTCTTCCCATT -3′; WT1 , Fwd: 5′- CCGCTATTCGCAATCAGGGT -3′, Rev: 5′- ACTTGTTTTACCTGTATGAGTCCTG -3′; AREG , Fwd: 5′- TGGATTGGACCTCAATGACA -3′, Rev: 5′- ACTGTGGTCCCCAGAAAATG -3′; EREG , Fwd: 5′- GCTCTGCCTGGGTTTCCATC -3′, Rev: 5′- CCACACGTGGATTGTCTTCTGTC -3′; CYCLIN E , Fwd: 5′- CTCCAGGAAGAGGAAGGCAA -3′, Rev: 5′- TCGATTTTGGCCATTTCTTCA -3′; GAPDH , Fwd: 5′- ACAGTCAGCCGCATCTTCTT -3′, Rev: 5′- ACGACCAAATCCGTTGACTC -3′. Western blotting and immunofluorescence analysis Western blotting analysis was performed as described before [40] . In brief, cells were incubated with non-denaturing lysis buffer (20 mM Tris HCl pH 8, 150 mM NaCl, 1% (v/v) NP-40, 2 mM EDTA) for 30 min and prepared for western blotting. Whole-cell lysates were electrophoresed and transferred to polyvinylidene difluoride membrane (Millipore). The membranes were blocked in PBS, 0.1% (v/v) Tween 20 and 5% (w/v) milk for 1 h at room temperature followed by incubation with primary antibodies (1:1,000 dilution) prepared in PBS, 0.1% (v/v) Tween 20 and 2.5% milk for 12 h at 4 °C. Membranes were then washed three times with PBS and incubated for 3 h with a horseradish peroxidase-conjugated anti-rabbit, anti-mouse or anti-goat IgG secondary antibody (1:5,000 dilution, Jackson ImmunoResearch). Membranes were washed three times with PBS and proteins were detected using ECL Western blotting detection kit (Amersham). Uncropped scans of western blottings are provided in Supplementary Figs 2–7 . Immunofluorescence analysis was performed as previously described [41] . Briefly, cells were grown on coverslips and were washed with PBS followed by cross-linking in 4% (v/v) paraformaldehyde in PBS for 15 min at room temperature. The cells were washed once in PBS and incubated in blocking solution for 30 min at room temperature. The cells were then incubated in PBS containing primary antibody (1:100 dilution) for 1 h and washed twice with PBS followed by incubation in DyLight 488- or DyLight 549-conjugated goat anti-rabbit/anti-mouse IgG secondary antibodies (1:500 dilution, Thermo Scientific) for 1 h. DNA was stained with Hoechst dye and the cells were mounted using Fluoromount-G (Southern Biotech). The immunofluorescence signal was visualized using Zeiss LSM 710 Confocal Microscope. The following antibodies were used for western blotting and immunofluorescence analysis: MAD2 (C-19-sc-6329, FL-205-sc-28261), CDC20 (sc-1907), CYCLIN B1 (sc-245), WT1-F6 (sc-7385) and WT1-C-19 obtained from Santa Cruz Biotechnology. MAD2 (A300-301A), MAD1 (A300-339A), BUBR1 (A300-386A), and CDC27 (A301-184A) antibodies were obtained from Bethyl Laboratories. SECURIN (ab3305), H3S10p (ab5176), H3 (ab1791), CENPA (ab13939) and β-TUBULIN (ab6046) antibodies were obtained from Abcam. APC/C-ubiquitination activity assay The APC/C-ubiquitination activity assay was performed as described before [20] . HeLa cells were blocked in prometaphase stage by treatment with 2.5 mM thymidine for 24 h, followed by treatment with 60 ng ml −1 nocodazole for 12 h. Nocodazole-arrested HeLa cells were washed with ice-cold PBS and resuspended in 75% of pellet volume of hypotonic buffer (20 mM Hepes-NaOH, pH 7.6, 5 mM KCl, 1 mM dithiothreitol) containing protease inhibitor cocktail (Roche). After repeated freeze-thawing on dry ice, the cell lysates were centrifuged at 13,000 r.p.m. for 1 h. The supernatant was supplemented with glycerol to 10% (v/v) and used in APC/C activity assay. Twenty-microlitre reaction mixtures contained 10 μl of concentrated mitotic extract (~ 10 mg ml −1 ), 2 μl of 10 × degradation mixture (100 mM Tris–HCl, pH 7.6, 50 mM MgCl 2 , 10 mM dithiothreitol, 10 mg ml −1 ubiquitin, 100 mM phosphocreatine, 5 mM ATP, 0.1 mg ml −1 UbcH10) and 1 μl of 20 × creatine phosphokinase (1 mg ml −1 ) (Sigma). Reactions were incubated at 30 °C in the presence of different recombinant proteins, and 3-μl samples were withdrawn at indicated time points in SDS–PAGE sample buffer. Degradation of CYCLIN B and SECURIN was followed by western blotting. How to cite this article: Shandilya, J. et al . WT1 interacts with MAD2 and regulates mitotic checkpoint function. Nat. Commun. 5:4903 doi: 10.1038/ncomms5903 (2014).